Chemical treatment enhances skipping of a mutated exon in thedystrophingene Duchenne muscular dystrophy (DMD) is a fatal muscle wasting disease caused by a loss of the dystrophin protein. Control of dystrophin mRNA splicing to convert severe DMD to a milder phenotype is attracting much attention. Here we report a dystrophinopathy patient who has a point mutation in exon 31 of the dystrophin gene. Although the mutation generates a stop codon, a small amount of internally deleted, but functional, dystrophin protein is produced in the patient cells. An analysis of the mRNA reveals that the mutation promotes exon skipping and restores the open reading frame of dystrophin. Presumably, the mutation disrupts an exonic splicing enhancer and creates an exonic splicing silencer. Therefore, we searched for small chemicals that enhance exon skipping, and found that TG003 promotes the skipping of exon 31 in the endogenous dystrophin gene in a dose-dependent manner and increases the production of the dystrophin protein in the patient's cells. Duchenne muscular dystrophy (DMD) is the most common inherited muscle disease and is caused by a mutation in the dystrophin gene, the largest in the human genome, on the X chromosome [1] . Because of progressive muscle wasting, DMD patients usually succumb to cardiac or respiratory failure in their twenties. Becker muscular dystrophy (BMD) is a milder allelic variant of DMD, usually affecting adult males. A reading frame rule explains the difference between DMD and BMD. Nonsense mutations or deletions causing frame shifts in the dystrophin mRNA, both of which create premature termination codons (PTCs), usually result in a severe DMD phenotype, because of a lack of the dystrophin protein. In contrast, mutations/deletions that maintain the original reading frame in the mRNA cause the milder BMD phenotype, as a mutated, but still functional, dystrophin protein can be expressed from the mRNA [2] . However, in some mild BMD cases, the patients had nonsense mutations in exons but still produced novel in-frame dystrophin mRNAs by skipping the exons containing the nonsense codon [3] , [4] , [5] , [6] , [7] . Thus, internally deleted but partially functional dystrophin proteins can be produced from the exon-skipped mRNAs. The current major therapeutic approach established by us, as well as by other groups, is to convert DMD to BMD phenotypes by restoring dystrophin protein expression by inducing exon skipping with antisense oligonucleotides (AONs) [8] , [9] , [10] , [11] . Several different AONs have been designed against either splice sites or splicing enhancer elements to induce exon skipping in cells of DMD patients. The AONs, which are designed to target those splicing elements, were demonstrated to restore the reading frame of dystrophin by causing skipping of the target exons. For example, the administration of an AON against an exonic splicing enhancer (ESE) in exon 19 promoted exon skipping in cells and increased production of an internally deleted dystrophin protein [12] , [13] , [14] . Another AON against exon 51 is currently under clinical trials [9] , [15] , [16] . However, considering the therapeutic cost and convenience, small chemical compounds have been highly awaited. A small compound PTC124 (refs 17 and 18 ), which induces read-through of the PTC, was reported to have the potential to treat some DMD patients who have nonsense mutations. Although a clinical trial of PTC124 for DMD patients who have nonsense mutations in the dystrophin gene was completed, no significant improvement of treated patients was observed ( http://www.ptcbio.com/May_DBMD_Trial_Update.htm ). We have been interested in the role of phosphorylation of SR proteins in splicing regulation. SR proteins are heavily phosphorylated in cells and are involved in constitutive and alternative splicing [19] , [20] . By extensive screening of 100,000 chemical compounds in a chemical library using in vitro phosphorylation assay, we identified several synthetic chemical compounds that inhibit SR protein kinases specifically. We first identified a synthetic compound as a specific inhibitor of SR protein kinases and named it as SRPIN340 (ref. 21 ). Administration of SRPIN340 to mice retina changed the splicing pattern of vascular endothelial growth factor-A and suppressed vascular generation [22] . We next identified TG003, a kinase inhibitor specific for Cdc-like kinases (Clks) [22] that are also able to phosphorylate SR proteins. TG003 affected splicing both in vitro and in vivo [23] , [24] . Recently, we reported that spliceostatin, originally characterized as an antitumour drug, blocked splicing and promoted the export of unspliced pre-mRNAs [25] , [26] . Here we tested these compounds to determine whether splicing in this context in ex vivo myoblast cell culture could be modified, and found that TG003 enhanced exon skipping and produced an internally deleted dystrophin protein in the in vitro -formed myotubes of a dystrophinopathy patient who has a point mutation in exon 31 of the dystrophin gene. Point mutation causes skipping of exon 31 in a DMD patient We have analysed and identified mutations in the dystrophin gene of more than 400 dystrophinopathy patients. We found that one patient (KUCG797) had a point mutation in exon 31. The mutation is a change from G to T (G to U on RNA) at position 4303 of the dystrophin cDNA (c.4303G>T, Fig. 1a ). As this change replaced GAG for glutamate with the TAG for a stop codon (p.Glu1435X), the patient was not expected to produce dystrophin, resulting in severe DMD. The immunostaining of a biopsied skeletal muscle, however, showed patchy and discontinuous signals with antibodies recognizing N- or C-terminal dystrophin domains ( Fig. 1e,f ), which are comparable to BMD. Size and shape of muscle fibres were heterogeneous. 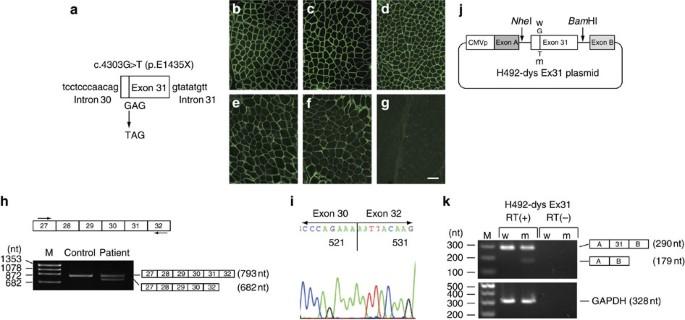Figure 1: Point mutation in exon 31 of thedystrophingene causes exon skipping and restores the open reading frame for an internally deleted protein. (a) A point mutation that was found in thedystrophingene of patient KUCG797. The position of c.4303G>T (p.Glu1435X) in exon 31 is indicated by the bar. (b–g) Dystrophin expression in the control (b–d) and in the patient's (e–g) muscles. Immunohistochemical examinations for C-terminal (DYS2), N-terminal (DYS3) and rod- (MANDYS1) domains were carried out. Immunoreactivity for DYS2 (exons 77–79 of dystrophin) and DYS3 (exons 10–12 of dystrophin) (e,f) was somewhat patchy and weaker in the patient's muscles as compared with the control cells (b,c). However, immunoreactivity for MANDYS1, which recognizes exon 31/32 of the dystrophin was defective only in the patient (compare panelsd,g). Scale bar, 50 μm. (h) The RT–PCR products obtained from the control and patient were analysed on agarose gels. The RT–PCR products from the patient's RNA contained an additional shorter product. The DNA sequences of these bands were analysed, and the structure of each PCR product is shown schematically at the right of the panel. (i) Sequencing of the shorter product seen in (c) confirmed the skipping of exon 31 in the patient. (j) A schematic representation of the hybrid minigene plasmids that harbour either the wild-type (W) or mutated (m) exon 31 of thedystrophingene. The minigene vector H492 encodes two cassette exons (A and B) and an intron sequence containing a multicloning site. Thedystrophingene region encompassing exon 31 with flanking introns was inserted into theNheI andBamHI sites in the intron region of H492. These plasmids were transfected into HeLa cells and the pre-mRNAs were transcribed from the cytomegalovirus (CMV) promoter (CMVp). (k) The RT–PCR products of wild-type (W) and mutant (m) mRNA that were recovered from transfected HeLa cells were visualized on agarose gel. Two different PCR products were detected only with H492-dys Ex31m plasmid. Glyceraldehyde-3-phosphate dehydrogenase (GAPDH) mRNA was used as a control for transfection efficiency. As negative controls, RT–PCR reactions without reverse transcriptase (RT−) were performed for both RNAs from the reporters and GAPDH. Figure 1: Point mutation in exon 31 of the dystrophin gene causes exon skipping and restores the open reading frame for an internally deleted protein. ( a ) A point mutation that was found in the dystrophin gene of patient KUCG797. The position of c.4303G>T (p.Glu1435X) in exon 31 is indicated by the bar. ( b – g ) Dystrophin expression in the control ( b – d ) and in the patient's ( e – g ) muscles. Immunohistochemical examinations for C-terminal (DYS2), N-terminal (DYS3) and rod- (MANDYS1) domains were carried out. Immunoreactivity for DYS2 (exons 77–79 of dystrophin) and DYS3 (exons 10–12 of dystrophin) ( e , f ) was somewhat patchy and weaker in the patient's muscles as compared with the control cells ( b , c ). However, immunoreactivity for MANDYS1, which recognizes exon 31/32 of the dystrophin was defective only in the patient (compare panels d , g ). Scale bar, 50 μm. ( h ) The RT–PCR products obtained from the control and patient were analysed on agarose gels. The RT–PCR products from the patient's RNA contained an additional shorter product. The DNA sequences of these bands were analysed, and the structure of each PCR product is shown schematically at the right of the panel. ( i ) Sequencing of the shorter product seen in ( c ) confirmed the skipping of exon 31 in the patient. ( j ) A schematic representation of the hybrid minigene plasmids that harbour either the wild-type (W) or mutated (m) exon 31 of the dystrophin gene. The minigene vector H492 encodes two cassette exons (A and B) and an intron sequence containing a multicloning site. The dystrophin gene region encompassing exon 31 with flanking introns was inserted into the Nhe I and Bam HI sites in the intron region of H492. These plasmids were transfected into HeLa cells and the pre-mRNAs were transcribed from the cytomegalovirus (CMV) promoter (CMVp). ( k ) The RT–PCR products of wild-type (W) and mutant (m) mRNA that were recovered from transfected HeLa cells were visualized on agarose gel. Two different PCR products were detected only with H492-dys Ex31m plasmid. Glyceraldehyde-3-phosphate dehydrogenase (GAPDH) mRNA was used as a control for transfection efficiency. As negative controls, RT–PCR reactions without reverse transcriptase (RT−) were performed for both RNAs from the reporters and GAPDH. Full size image To explain the discrepancy between the genotype and the immunostaining pattern, we presumed that the nonsense mutation in exon 31 disrupted the ESE, which resulted in skipping of the mutated exon in the patient's muscle cells. To test this possibility, we analysed the dystrophin mRNA in skeletal muscle. The reverse transcription polymerase chain reaction (RT–PCR) amplification of the region extending from exon 27 to exon 32 showed two nearly equal amounts of two products: one of expected size with exons 27–32, including the TAG stop codon in exon 31, and the other a smaller product lacking exon 31 ( Fig. 1h,i ). However, the other introns of this dystrophin gene, which consists of 79 exons, seemed to be correctly spliced out ( Supplementary Fig. S1 , (−) lanes and Supplementary Table S1 ). The resulting dystrophin mRNA lacking the 111-bp-long exon 31 was in-frame to produce an internally deleted, but likely functional, dystrophin protein. In the patient's muscle cells, the exon 31-containing mRNA should be lost by NMD, and only the internally deleted protein transcribed from the exon 31-skipped transcript can be expressed. Therefore, the dystrophin protein was immunostained with antibodies against the N- or C-terminal domains of dystrophin ( Fig. 1b,c,e,f ), but failed to be recognized by MANDYS1, a monoclonal antibody against the exon 31-encompassing region in the patient's cells ( Fig. 1d,g ). Splicing regulators involved in exon 31 splicing These results suggest that the point mutation in exon 31 not only produces a stop codon but also modifies an exonic splicing regulatory site. To test this hypothesis, we incorporated the wild-type and mutant dystrophin gene fragment that retains exon 31 and the flanking introns into the H492 vector, which has been used for splicing analysis in cells ( Fig. 1j ) [27] , [28] , [29] , and transfected them into HeLa cells. Two PCR products were detected with the mutant plasmid ( Fig. 1k ), whereas only a single RT–PCR product was amplified from the wild-type plasmid. Sequencing analysis revealed that the smaller PCR product from the mutant does not include exon 31 (data not shown). As mutant exon 31 with flanking introns cloned into the H492 vector is sufficient to promote skipping, we tried to identify the splicing regulatory factors that bind to the RNA portion. According to the SpliceAid program ( http://www.introni.it/splicing.html ) [30] , exon 31 has the binding sequence of SRp30c/SRSF9 identified by SELEX ( Supplementary Fig. S2b ) [31] . The point mutation found in the patient disrupts the binding site of SRp30c/SRSF9, a member of the SR protein family ( Supplementary Fig. S2a ), which are often purine-rich and known to bind to ESEs. In addition, the mutation presumably generates an RNA sequence that has high homology to exonic splicing silencers (ESSs) recognized by the heterogeneous nuclear ribonucleoproteins (hnRNPs) A1 ( Supplementary Fig. S2a,b ) [32] . To test this notion, we first compared the binding to hnRNP A1 of the mutant RNA with that of the wild-type RNA in a gel mobility shift assay. The recombinant hnRNP A1 was prepared as a glutathione S -transferase (GST)-tagged protein ( Supplementary Fig. S3b , lane 3) and mixed with either the wild-type or mutant dystrophin RNA, and the resultant complexes were analysed by native polyacrylamide gel electrophoresis. 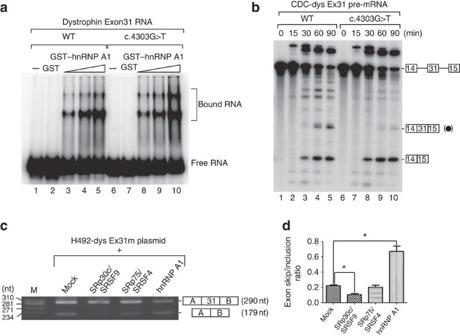Figure 2: The point mutation in exon 31 enhances binding to hnRNP A1 and exon skipping bothin vitroandin vivo. (a) Gel mobility shift assays with GST–hnRNP A1 and dystrophin exon 31 RNA.32P-labelled dystrophin exon 31 RNA (wild type or mutant) was incubated with either GST alone (GST: lanes 2 and 7, 400 ng) or with GST-tagged hnRNP A1 (GST–hnRNP A1: lanes 3–5 and 8–10; 100, 200 and 400 ng, respectively), and the resultant complexes were subjected to 8% native polyacrylamide gel electrophoresis. Lanes 1 and 6 show where RNA itself migrates on the gel (marked as Free RNA on the right of the panel). Complexes of hnRNP A1 and RNA are also indicated as Bound RNA. All incubations were carried out at 20 °C for 30 min. (b)In vitrosplicing assays with pre-mRNAs that contain exon 31.32P-labelled chicken δ-crystallin (CDC) pre-mRNA containing either wild-type (WT) or mutant (c.4303G>T) exon 31 in the intron was incubated with HeLa cell nuclear extracts at 30 °C for the time shown at the top of the panel. The RNA products were analysed by electrophoresis on 6% denaturing gel. The structures of the pre-mRNA and two different mRNAs are shown at the right of the panel. Boxes with numbers indicate exons, whereas the lines between boxes designate introns. The mRNA that includes exon 31 (closed circle) was produced more efficiently with CDC-dys Ex31 WT pre-mRNA than CDC-dys Ex31 c.4303G>T pre-mRNA. (c) Effect of overexpression of several RNA-binding proteins on the inclusion and skipping of the mutant exon 31. HeLa cells (3×106cells) were cultured overnight and transfected with 150 ng of the mutant reporter plasmid used inFigure 1fin combination with 1.5 μg of the plasmid that expresses designated proteins with a Flag tag. RNAs were recovered and analysed by RT–PCR. The skipping of the mutated exon 31 was inhibited by SRp30c/SRSF9, but promoted by hnRNP A1. (d) Quantification of the ratio between exon skipping and inclusion for the RNA expressed from the mutant reporter plasmid in the presence of several RNA-binding proteins. Averages and standard deviations from three independent experiments are shown. *P<0.005. As shown in Figure 2a , two hnRNP A1–RNA complexes showed different patterns of migration on the gel (lanes 3–5 and 8–10). The faster-migrating complex contains one hnRNP A1 molecule on the RNA probe, whereas the slower-migrating complex includes more than two hnRNP A1 molecules [33] . The faster-migrating complex could be detected with both the wild-type and mutant RNA even at a low concentration of GST–hnRNP A1 (lanes 3 and 8), reflecting the efficiency of its formation with either RNA at the hnRNP A1-binding site conserved in exon 31 (ref. 5 ). In contrast, the slower-migrating complex was formed two times more efficiently with the mutant than with wild-type RNA at each concentration of GST–hnRNP A1 protein (compare lanes 3–5 and 8–10), and the difference was most obvious at the highest protein concentration (0.5 μM; lanes 5 and 10). As the estimated hnRNP A1 protein concentration in the HeLa nucleus is ~145 μM (hnRNP A1 6–7×10 7 molecules per cell [34] , [35] , and 690 μm 3 for the volume of the HeLa cell nucleus [36] ), the second binding site of the mutant exon 31 would be occupied by hnRNP A1 in vivo . As a control, GST alone was used for the assays and no binding was detected ( Fig. 2a , lanes 2 and 7). Figure 2: The point mutation in exon 31 enhances binding to hnRNP A1 and exon skipping both in vitro and in vivo . ( a ) Gel mobility shift assays with GST–hnRNP A1 and dystrophin exon 31 RNA. 32 P-labelled dystrophin exon 31 RNA (wild type or mutant) was incubated with either GST alone (GST: lanes 2 and 7, 400 ng) or with GST-tagged hnRNP A1 (GST–hnRNP A1: lanes 3–5 and 8–10; 100, 200 and 400 ng, respectively), and the resultant complexes were subjected to 8% native polyacrylamide gel electrophoresis. Lanes 1 and 6 show where RNA itself migrates on the gel (marked as Free RNA on the right of the panel). Complexes of hnRNP A1 and RNA are also indicated as Bound RNA. All incubations were carried out at 20 °C for 30 min. ( b ) In vitro splicing assays with pre-mRNAs that contain exon 31. 32 P-labelled chicken δ-crystallin (CDC) pre-mRNA containing either wild-type (WT) or mutant (c.4303G>T) exon 31 in the intron was incubated with HeLa cell nuclear extracts at 30 °C for the time shown at the top of the panel. The RNA products were analysed by electrophoresis on 6% denaturing gel. The structures of the pre-mRNA and two different mRNAs are shown at the right of the panel. Boxes with numbers indicate exons, whereas the lines between boxes designate introns. The mRNA that includes exon 31 (closed circle) was produced more efficiently with CDC-dys Ex31 WT pre-mRNA than CDC-dys Ex31 c.4303G>T pre-mRNA. ( c ) Effect of overexpression of several RNA-binding proteins on the inclusion and skipping of the mutant exon 31. HeLa cells (3×10 6 cells) were cultured overnight and transfected with 150 ng of the mutant reporter plasmid used in Figure 1f in combination with 1.5 μg of the plasmid that expresses designated proteins with a Flag tag. RNAs were recovered and analysed by RT–PCR. The skipping of the mutated exon 31 was inhibited by SRp30c/SRSF9, but promoted by hnRNP A1. ( d ) Quantification of the ratio between exon skipping and inclusion for the RNA expressed from the mutant reporter plasmid in the presence of several RNA-binding proteins. Averages and standard deviations from three independent experiments are shown. * P <0.005. Full size image Consistent with the low binding score for SRp30c predicted by a Splice Aid analysis, weak binding of the SRp30c protein to the wild-type RNA was detected in the gel mobility shift assay ( Supplementary Fig. S3a , lanes 3–5). However, the binding of SRp30c to the mutated RNA was 25–50% lower than that to the wild type (lane 8–10), indicating that the point mutation of exon 31 affects the recognition by SRp30c. All the results described above strongly suggested that the mutated exon 31 was not efficiently recognized as an exon in the context of splicing. To confirm this, we carried out in vitro splicing assays. For the assays, we prepared pre-mRNA that contains either the wild-type or mutant exon 31 in the intronic region of chicken δ-crystallin (CDC) pre-mRNA [37] ( Fig. 2b ). The production of spliced mRNA containing the wild-type exon 31 (black circle) was detected with CDC-dys Ex31w pre-mRNA after a 60-min incubation ( Fig. 2b , lanes 3–5). In contrast, the production of mRNA containing exon 31 from the CDC-dys Ex31m pre-mRNA was suppressed ( Fig. 2b , lanes 8–10). Next we investigated the effect of the overexpression of these RNA-binding proteins on the splicing pattern of a minigene in HeLa cells. As shown in Figure 1f previously, this minigene produced mRNA both with and without exon 31 ( Fig. 2c , mock). When SRp30c/SRSF9 was overexpressed, the rate of exon skipping was reduced ( Fig. 2c,d , SRp30c/SRSF9). In contrast, overexpression of hnRNP A1 promoted exon skipping ( Fig. 2c,d , hnRNP A1, and Supplementary Fig. S4a ). Although hnRNP A1 is an abundant protein in HeLa cells, as mentioned previously, we could detect similar amount of the exogenous protein to that of the endogenous protein ( Supplementary Fig. S4b ). As a control, SRp75/SRSF4, another SR protein [38] , was used for the same assay, but failed to change the splicing pattern ( Fig. 2c,d , SRp75/SRSF4). These results indicated that the skipping of the exon 31 in the dystrophin RNA was promoted by disruption of the SRp30c/SRSF9-dependent ESE and production of an hnRNP A1-dependent ESS in exon 31. TG003 promotes skipping of a mutated exon 31 in HeLa cells The fact that this patient can express an internally deleted but presumably partially functional dystrophin protein made us look for chemical compounds that promote the skipping of exon 31 for further production of the internally deleted protein to improve the patient's condition. We screened for specific inhibitors of a variety of kinases and found several compounds that affect alternative splicing [21] . As these chemicals were demonstrated to affect alternative splicing in vitro and in vivo , we investigated the effect of eight compounds on the mutated exon 31 using the H492 minigene vector ( Supplementary Table S2 ). TG003 strongly induced the skipping of the mutated exon in comparison with SRPIN340 and the solvent alone ( Fig. 3a,b , dimethylsulphoxide, TG003 and SRPIN340). To examine the effect of TG003 on the wild-type exon 31, we next incubated cells with different concentrations of the compound after transfection of the minigene plasmids. 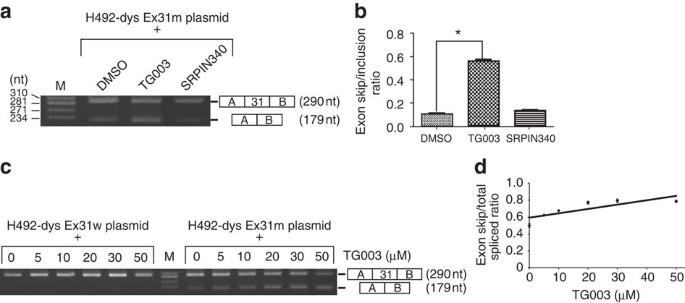Figure 3: TG003 promotes skipping of mutated exon 31 in HeLa cells in a dose-dependent manner. (a) Effect of chemical compounds on exon 31 skipping with a heterologous reporter construct in HeLa cells. After transfection of the reporter plasmid (H492-dys Ex31m) as given inFigure 2c, HeLa cells were incubated in the presence of the chemical compounds at 30 μM for 24 h. Dimethylsulphoxide (DMSO) was used as a negative control as it was used as a solvent of compounds. RNAs were recovered and analysed by RT–PCR. TG003, but not SRPIN340, promoted skipping of the mutated exon 31. (b) Quantification of the ratio between exon skipping and inclusion for the RNA products expressed from the mutant reporter plasmid in the presence of several RNA-binding proteins. Averages and standard deviations from three independent experiments are shown. *P<0.0001. (c) RT–PCR of the RNA recovered from the reporter plasmid-transfected HeLa cells cultured in the presence of several concentrations of TG003. (d) Quantification of the ratio of exon skipping to total spliced for the RNA products expressed from the mutant reporter plasmid in the presence of several concentrations of TG003 by quantitative RT–PCR. Averages and standard deviations from three independent experiments are shown. As shown in Figure 3c , TG003 promoted the skipping of the mutated exon 31 in a dose-dependent manner ( Fig. 3c ), but did not affect splicing of the wild type even at 50 μM ( Fig. 3c ). By quantitative RT–PCR analysis, we found that the ratio of skipped mRNA to total spliced mRNAs was increased by TG003 in a dose-dependent manner ( Fig. 3d ). We then looked for other patients who were sensitive to TG003, and found one patient whose mutated exon was skipped on the administration of TG003 ( Supplementary Fig. S5 ). This dystrophy patient has a point mutation in exon 27 (c.3613delG (p.Glu1205LysfsX9)), which produces a premature termination codon via a frameshift. We cloned the dystrophin gene fragment containing the mutant exon 27 and flanking introns into the H492 vector and transfected the plasmid into HeLa cells. As shown in Supplementary Figure S5 , exon 27-skipped mRNA production was promoted by TG003 in a dose-dependent manner with the mutant plasmid in HeLa cells, whereas splicing of the wild-type mRNA was not affected. Figure 3: TG003 promotes skipping of mutated exon 31 in HeLa cells in a dose-dependent manner. ( a ) Effect of chemical compounds on exon 31 skipping with a heterologous reporter construct in HeLa cells. After transfection of the reporter plasmid (H492-dys Ex31m) as given in Figure 2c , HeLa cells were incubated in the presence of the chemical compounds at 30 μM for 24 h. Dimethylsulphoxide (DMSO) was used as a negative control as it was used as a solvent of compounds. RNAs were recovered and analysed by RT–PCR. TG003, but not SRPIN340, promoted skipping of the mutated exon 31. ( b ) Quantification of the ratio between exon skipping and inclusion for the RNA products expressed from the mutant reporter plasmid in the presence of several RNA-binding proteins. Averages and standard deviations from three independent experiments are shown. * P <0.0001. ( c ) RT–PCR of the RNA recovered from the reporter plasmid-transfected HeLa cells cultured in the presence of several concentrations of TG003. ( d ) Quantification of the ratio of exon skipping to total spliced for the RNA products expressed from the mutant reporter plasmid in the presence of several concentrations of TG003 by quantitative RT–PCR. Averages and standard deviations from three independent experiments are shown. Full size image TG003 promotes dystrophin expression in the patient's cells As the results obtained with a minigene construct strongly suggested that TG003 could induce exon 31-specific skipping, we next examined the effect of TG003 on splicing of the dystrophin gene in myoblasts. Muscle cells obtained from the patient were cultured on dishes. Equivalent amounts of dystrophin mRNA with and without exon 31 were detected by RT–PCR ( Fig. 4a ). When TG003 was added to these cells, it was shown by quantitative RT–PCR analysis that the ratio of exon 31-skipped mRNA to total mRNAs was increased in a concentration-dependent manner ( Fig. 4b ). To examine the effect of TG003 on the splicing of other dystrophin introns, we prepared a subset of primers to amplify all 79 exons of dystrophin . The results of RT–PCR with or without TG003 showed that all exons except exon 31 were included ( Supplementary Fig. S1 and Supplementary Table S1 ), indicating that TG003 selectively promotes skipping of the mutated exon 31 in the patient's cells (or a mutated exon 27 in another patient). 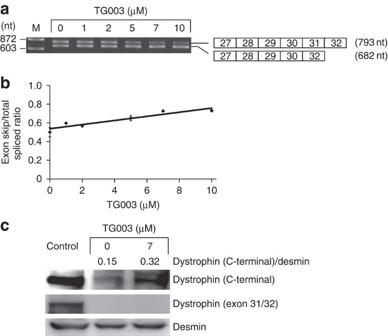Figure 4: TG003 induces not only exon 31 skipping but also Δexon 31 dystrophin protein expression in patient cells. (a) RT–PCR with RNA recovered from primary cultured muscle cells treated with different amounts of TG003. (b) Quantification of the ratio of exon skipping to total spliced for the RNA products expressed from the patient's endogenousdystrophingene by quantitative RT–PCR. Averages and standard deviations from three independent experiments are shown. (c) Western blotting of dystrophin protein expression in TG003-treated cells. Proteins were detected with antibodies recognizing either the C terminus of dystrophin or the peptide encoded by exon 31. The antibody against desmin indicated that equivalent numbers of the cells were used for this assay. Figure 4: TG003 induces not only exon 31 skipping but also Δexon 31 dystrophin protein expression in patient cells. ( a ) RT–PCR with RNA recovered from primary cultured muscle cells treated with different amounts of TG003. ( b ) Quantification of the ratio of exon skipping to total spliced for the RNA products expressed from the patient's endogenous dystrophin gene by quantitative RT–PCR. Averages and standard deviations from three independent experiments are shown. ( c ) Western blotting of dystrophin protein expression in TG003-treated cells. Proteins were detected with antibodies recognizing either the C terminus of dystrophin or the peptide encoded by exon 31. The antibody against desmin indicated that equivalent numbers of the cells were used for this assay. Full size image Therefore, we next examine whether TG003 really increases the expression of the internally deleted, but functional, dystrophin protein in the patient's cells. Western blotting with an antibody that specifically recognizes the C terminus of dystrophin showed that the administration of TG003 (7 μM) increased the protein expression ( Fig. 4c ). The ratio of dystrophin (C terminal) signal to desmin signal was increased more than double by TG003. The antibody specific for the peptide with exon 31 did not detect it, indicating that the dystrophin protein lacks an exon 31-coding peptide ( Fig. 4c ). Therefore, TG003 promoted the expression of an internally deleted dystrophin protein by inducing exon 31 skipping in cells derived carrying the c.4303G>T mutation. This paper describes a patient with dystrophinopathy who had a point mutation in exon 31 of the dystrophin gene. As the mutation creates an in-frame stop codon, the mRNA was not expected to produce a protein. However, RT–PCR demonstrated that exon 31 was skipped and the dystrophin mRNA was naturally generated in this patient, and an internally deleted dystrophin protein was produced ( Fig. 1e–g ). We found that the point mutation in exon 31 disrupted the SRp30c-mediated ESE, and simultaneously created an ESS bound to hnRNP A1. This case is similar to that of the survival of motor neuron 2 ( SMN2 ) gene [39] , [40] , [41] , [42] . The SMN2 gene has a C/T transition compared with the SMN1 gene, which results in prevention of efficient exon 7 splicing. In these cases, either mutations or polymorphisms in exons can affect splicing by disrupting a positive element and creating a negative element [39] , [40] , [41] , [42] . In addition to affecting ESE, the c.4303G>T mutation increased the number of hnRNP A1-binding sites in exon 31 of the dystrophin gene. There was already one hnRNP A1-binding site in exon 31, but this mutation added another. The hnRNP A1 protein was shown to bind RNA cooperatively [43] , and this would be facilitated by two high-affinity binding sites [44] . In our case, the hnRNP A1-cooperative binding seems to be facilitated by the c.4303G>T mutation, affecting the recognition and skipping of exon 31, as shown in Figure 2 . It is very likely that there are more diseases and mutant phenotypes caused by the disruption/creation of splicing elements, as alternative splicing is maintained by a balance of positive and negative cis -elements in conjunction with trans factors. Our results demonstrated that TG003 promoted exon skipping only in the mutant exon 31, but not in the wild type. TG003 is a specific inhibitor for Clks [23] , and Clks have been shown to phosphorylate SR proteins [24] , [45] , [46] , [47] , [48] . SRp30c/SRSF9 is likely involved in the recognition of exon 31 for splicing ( Fig. 2 and Supplementary Figs S2 and S3 ) and can be a target of TG003. However, TG003 had no effect on the splicing of the wild-type exon 31, in which SRp30c/SRSF9 is involved ( Fig. 3c ). We assume that SRp30c contributes to the inclusion of the exon, but it is not phosphorylated by Clk in the nucleus. Therefore, TG003 had no effect on WT exon 31. Moreover, we have currently demonstrated that the overexpression of Clks results in the specific phosphorylation of SRp75/SRSF4 among SR proteins in vivo [24] . This means that not all SR proteins are phosphorylated by Clks. It has been reported that the roles of SR proteins in splicing are not always the same. Although it is generally assumed that SR proteins promote the inclusion of exons, some SR proteins can cause the skipping of exons in several alternative splicing events [19] , [20] , [49] . Thus, it is possible that some SR protein(s), which is phosphorylated by Clks, remains dephosphorylated by TG003, and this protein cooperates with hnRNP A1 as a coinhibitor of the recognition of exon 31 during splicing. Another possibility is that hnRNP A1 is a specific target of Clks, although there has been no evidence for this. Further experiments are required to examine these possible scenarios. In this patient, skipping of the mutated exon 31 restores the open reading frame. Therefore, it is likely that an internally deleted, but functional, dystrophin protein is expressed ( Fig. 1e–g ). This strongly suggests that better clinical features could be expected if the skipping is induced more efficiently to produce more of the internally deleted protein. We found that TG003, reported as a Clk-specific inhibitor, stimulated skipping of the exon in both a minigene construct and the endogenous pre-mRNA in the patient's cells. When we administered 10 μM of TG003 into HeLa and COS cells, no morphological changes were observed and growth rate was not affected up to 3 days [23] . We also confirmed that TG003 had no cytotoxicity in HeLa cells at the dosage used in Figure 3c (data not shown), and even in mice at up to 100 mg kg −1 per day per os (Onogi H. and Hagiwara M., unpublished data). As shown in Figure 3c , TG003 induced the skipping of the mutated exon 31, but did not affect the splicing of the wild type. The selectivity of the effect of TG003 may explain the weak toxicity of the compound. TG003 was recently shown to inhibit the replication of the influenza virus by modifying the processing of viral RNA in cells [50] . Although more preclinical studies with animal models are needed, TG003 is the first chemical compound that is verified to improve dystrophin production in in vitro patient-derived myotubes. We thus started to look for patients sensitive to TG003, and found another dystrophy patient whose mutated exon was skipped ( Supplementary Fig. S5 ). We hope that our findings will contribute towards the development of a therapy of Duchenne muscular dystrophy. Case The proband (KUCG 797) was a 5-year-old boy born to healthy Japanese parents without any family history of muscle disease. He started to walk independently at 1 year and 4 months of age and his motor development was normal. At the age of 2 years, his serum creatine kinase level was found to be 2,567 IU l −1 (normal <169 IU l −1 ) in a routine blood examination conducted on admission to hospital. He was referred to Kobe University Hospital to have his dystrophin gene examined for mutations. The mild creatine kinase elevation persisted (1,331–4,740 IU l −1 ). No muscle weakness or abnormal gait was observed. At the age of 5 years, a muscle biopsy was performed. Informed consent for all study aspects including genetic testing was obtained from the parents, and these studies were approved by our ethics committees. Mutation analysis DNA was isolated from blood samples by standard phenol–chloroform extraction methods. Total RNA was isolated from peripheral lymphocytes that were collected from whole blood using Ficoll–Paque density gradients (Amersham Biosciences AB) or from thin-sliced muscle sections of frozen muscle samples. RT–PCR and RT-nested PCR were used to analyse the dystrophin mRNA expressed in skeletal muscle. A region encompassing exons 27–32 was amplified using an inner set of primers (forward c27f and reverse 2F, Supplementary Table S1 ). The products were purified and sequenced either directly or after subcloning into the vector pT7 Blue-T (Novagen). The DNA sequences were determined using an automated DNA sequencer (model 310; Applied Biosystems). Plasmid construction To construct H492-dys Ex31w and H492-dys Ex31m, the fragments encompassing exon 31 and flanking intronic regions were amplified from the genomic DNA of both the control and the patient by PCR. The primers used were Int 30f- Nhe I: 5′-GCGGCTAGCGTGATCCACCTGCCTCGAC-3′ and Int 31r- Bam HI: 5′-GCGGGATCCTCAAATCCAATCTTGCCAAT-3′. The amplified products were digested with Nhe I and Bam HI (New England Biolabs), and inserted into the H492 that had been digested with the same restriction enzymes. For the construction of Flag-SRp30c and Flag-SRp75, PCR-amplified human SRp30c and mouse SRp75 cDNAs were inserted between the Bam HI site and Xho I site of Flag-pCDNA3 (ref. 51 ), respectively. Human hnRNP A1 cDNA was amplified by PCR and inserted between the Bam HI and Not I sites of Flag-pCDNA3 (ref. 52 ) to construct Flag-hnRNP A1. To construct template plasmids for gel mobility shift assays, PCR-amplified wild-type and mutant dystrophin exon 31 were cloned into the Hin dIII and Xho I sites of pCDNA3 (Invitrogen). The resultant plasmids were designated as pCDNA3–dys Ex31w and pCDNA3–dys Ex31m. For making pCDC–dys Ex31w and pCDC–dys Ex31m, the wild-type or mutant exon 31 of the dystrophin gene was amplified by PCR and inserted between Sac I and Sty I sites of pCDC [37] . For protein expression in Escherichia coli , cDNAs for hnRNP A1 and SRp30c/SRSF9 lacking their termination codons were PCR-amplified and cloned between the Bam HI and Xho I sites of pET-GSTII [53] . All plasmids described above were verified by sequencing. Cell culture and transfection HeLa cells were cultured as described previously [37] . Transfection of the plasmids was carried out by using Lipofectamine 2000 as recommended by the manufacturer. After 24 h of transfection, RNAs were recovered from the transfected cells. The chemical compounds were incubated for 24 h. Primary culture of the DMD patient's muscle cells The patient's muscle cells were cultured in DMEM (Sigma) supplemented with 20% fetal bovine serum (Gibco), 4% Ultrocer G (PALL) and 1% antibiotic-antimycotic (Gibco) in a six-well plate (gelatin-coated micro plate (six-well) with lid, IWAKI) until confluent. To induce their differentiation into myotubes, the cells were cultured in DMEM (Sigma) supplemented with 2% horse serum (Gibco) and 1% antibiotic-antimycotic (Gibco) for 2 weeks with or without TG003. The medium and TG003 were refreshed every 2 days. Immunonohistochemical analyses of skeletal muscle Skeletal muscle samples obtained from the rectus muscle of the thigh by biopsy were flash-frozen with isopentane cooled in liquid nitrogen. Serial 10-μm-thick frozen sections were analysed with histochemical staining. The procedure for the immunohistochemistry was as follows: serial 10-μm-thick frozen muscle sections were fixed in cold acetone for 5 min. After blocking with normal goat serum, sections were incubated with primary antibodies overnight at 4 °C. The antibodies used were antidystrophin (DYS2: recognizing an epitope in exons 77–79, and DYS3: recognizing an epitope in exons 10–12, Novocastra) and antidystrophin (MANDYS1: recognizing an epitope in exon 31/32, a gift from Professor Dr Glenn E. Morris). After six rinses with PBS, sections were incubated with secondary antibodies, Alexa Fluor 488-labelled goat anti-mouse or anti-rabbit antibodies, at room temperature for 90 min. Isolation of RNA and RT–PCR RNA was isolated and analysed by RT–PCR, as described previously [4] . Primers used for amplification of dystrophin and human glyceraldehyde-3-phosphate dehydrogenase mRNAs are demonstrated in Supplementary Table S1 . PCR products were analysed on 2% agarose gels in Tris–borate/EDTA buffer. Skipping efficiencies were determined from gel images by comparing the shortened dystrophin mRNAs to the intact transcript of full length in a densitometric analysis with Image J software (for patient samples) or by quantifying the skipped products with a DNA 1000 LabChip Kit on an Agilent 2100 bioanalyzer (Agilent Technologies; for hDMD mouse samples). Exon skip/inclusion ratios were calculated as the amount of skipped transcript relative to the full-length transcript. Where appropriate, a two-tailed Student's t -test was used to determine the statistical significance of the skipping. As DNA size markers, φX174- Hae III digest (TAKARA) or 2-Log DNA ladder (New England Biolab) was used for agarose gel electrophoresis. Quantitative real-time RT–PCR Real-time RT–PCR amplification was performed using a 7500 fast real-time PCR system (Applied Biosystems Inc.). Real-time PCR assays were carried out in a final volume of 20 μl consisting of 10 μl of TaqMan Fast Advanced Master Mix (Applied Biosystems Inc.), 18 pmol each of 5′ and 3′ primer, 5 pmol of specific probe and 10 ng of the sample cDNA. The real-time PCR conditions were as follows: 1 cycle for 20 s at 96 °C, followed by 40 cycles of 2 s at 96 °C for denaturation, 15 s at 60 °C for annealing and 15 s at 72 °C for extension. Spectral data were captured and analysed using 7500 Real-Time Analysis Software version 2.0.3 (Applied Biosystems Inc.). All samples were run in triplicate. β-Actin and desmin was analysed as an endogenous RNA reference gene for normalization of H492-dys 31-derived mRNA and endogenous dystrophin mRNA from the patient, respectively. Exon skip/total ratios were calculated as the proportion of skipped transcript relative to both the full-length and the skipped transcripts. The PCR primers and probes (5-FAM and 3-MGB) were designed with Primer Express software (Applied Biosystems Inc.), and the sequences of the primers and probes are shown in Supplementary Table S1 . Western blotting with the patient's myotubes The patient's myotube cells were rinsed twice with PBS and then collected using 1× Cell Lysis Buffer (Cell Signaling Technology). Total protein (60 μg) was loaded on a 3–10% gradient polyacrylamide gel (PAGEL, ATTO). The fractionated proteins were transferred to HYBOND-P (GE Healthcare). Western blotting was performed using the ECL advance Western Blotting Detection kit (GE Healthcare) according to the manufacturer's instructions. The membrane was incubated with an antibody against the C terminus (NCL-DYS2, Leica) and exon 31 (MANDYS8, a gift from Dr Glenn E. Morris) of dystrophin at a dilution of 1:10 and 1:100, respectively. The dystrophin–antidystrophin immune complexes were detected with anti-mouse IgG (GE Healthcare). Western blotting for desmin was performed using the same protocol as described above. The Desmin antibody (H-76, Santa Cruz) was used at a dilution of 1:50. The desmine–antidesmine immune complexes were detected with anti-rabbit IgG (GE Healthcare). Preparation of recombinant proteins All proteins were overexpressed in BL21 (DE3) CodonPlus-RIPL cells (Stratagene). GST-His, GST-hnRNP A1-His and GST-SRp30c-His were induced at 20 °C overnight, purified according to the manufacturer's instructions (Pharmacia) and dialysed against PBS. Dialysed proteins were further purified on nickel resin (Qiagen) as recommended by the manufacturer and dialysed against buffer E (20-mM HEPES-KOH pH 7.9, 100-mM KCl, 0.2-mM EDTA, 10% glycerol and 1-mM DTT). Purified proteins were quickly frozen by liquid nitrogen and stored at −80 °C. In vitro transcription and splicing assay As templates, pCDNA3–dys Ex31 and pCDNA3–dys Ex31m were linearized with Xho I, and pCDC–dys Ex31w and pCDC–dys Ex31m were linearized with Sma I. In vitro transcription and purification of the transcribed RNAs were performed as described previously [37] . HeLa cell nuclear extracts were obtained from Cilbiotech. In vitro splicing assay was carried out in a 10-μl scale as described previously [37] . The RNAs were analysed by 6% denaturing polyacrylamide gel electrophoresis and autoradiography. Gel mobility shift assay Gel mobility shift assays were essentially carried out as described previously [54] . The binding buffer that was used contained 16-mM HEPES-KOH (pH 7.9), 80-mM KCl, 0.16-mM EDTA, 0.8-mM DTT, 8% glycerol, 100 ng μl −1 of BSA, 50 ng μl −1 of E. coli tRNA (Sigma Chemical Co.), 5×10 4 c.p.m. of RNA (dystrophin exon 31 wild type or mutant RNA) and 1 U μl −1 of RNasin (Promega). Eight percent native polyacrylamide gels were used to analyse the complexes. Statistical analyses Statistical analyses were performed with Prism5 statistical software (GraphPad) using a paired t -test or a one-way analysis of variance, followed by Tukey's multiple comparison test. How to cite this article: Nishida, A. et al . Chemical treatment enhances skipping of a mutated exon in the dystrophin gene. Nat. Commun. 2:308 doi: 10.1038/ncomms1306 (2011).